Heterothermy in growing king penguins A drop in body temperature allows significant energy savings in endotherms, but facultative heterothermy is usually restricted to small animals. Here we report that king penguin chicks ( Aptenodytes patagonicus ), which are able to fast for up to 5 months in winter, undergo marked seasonal heterothermy during this period of general food scarcity and slow-down of growth. They also experience short-term heterothermy below 20 °C in the lower abdomen during the intense (re)feeding period in spring, induced by cold meals and adverse weather. The heterothermic response involves reductions in peripheral temperature, reductions in thermal core volume and temporal abandonment of high core temperature. Among climate variables, air temperature and wind speed show the strongest effect on body temperature, but their effect size depends on physiological state. The observed heterothermy is remarkable for such a large bird (10 kg before fasting), which may account for its unrivalled fasting capacity among birds. In response to nutritional or climatic constraints, many small mammals and birds save energy by reducing heat production and allowing a temporary decline in body temperature ( T b ). States of hibernation and torpor are at the extreme end of heterothermic responses to environmental constraints, with the largest bird known to employ torpor weighing 500 g (refs 1 , 2 ). There is less scope for heterothermy in larger endotherms given that cooling and rewarming rates are size dependent [3] . Accordingly, during periods of food shortage large birds usually rely on their body stores and behavioural thermoregulatory mechanisms. For example, emperor penguins ( A. forsteri ) huddle together during their 4-month breeding fast, and maintain daily mean body temperatures in the abdomen within a narrow range of 1–2 °C of normothermic levels at around 37.5 °C (ref. 4 ). Similarly, although adult king penguins are known to tolerate heterothermy during deep foraging dives at sea, they apparently do not exhibit notable heterothermy during long-term fasts ashore [5] , [6] . Growing king penguin chicks, while only 3–4 months old, experience a severe nutritional bottleneck, when parental food provisioning is irregular and scarce or may cease altogether during the austral winter. Remarkably, experimentally deprived chicks showed a fasting endurance for up to 5 months, which, among birds, is unrivalled [7] . Young king penguins wear a downy plumage for a period of 10 months, but they achieve thermal independence at 1 month from hatch [8] . Left alone by their parents and living off their body stores, chicks aggregate into crèches. However, these comprise only loose aggregations compared with the tight huddles formed by emperor penguins. At the end of the winter season, parents feed their single chick more frequently, which replenishes its energy stores, notably subcutaneous fat, before its first moult into a waterproof plumage [9] . Although fasting chicks can tolerate the loss of up to 74% of their energy stores [10] , a high percentage of them run short of fuel before the end of winter [9] . Thus, saving energy during fasting periods becomes a matter of life or death. Adult king penguins are known to adapt to long-term fasts ashore by reducing their metabolism and protein catabolism within few days after beginning their fast, when body stores are still abundant [11] . King penguin chicks also display this protein-sparing physiology [7] , [10] , [12] and, moreover, slow down structural growth during winter [13] . The adaptive significance of these induced responses (after Schew and Ricklefs [14] ) to food shortage is presumably enhanced survival while relying on endogenous energy stores and by deferring maturation (fledgling) and, thus, self-reliance to a time of higher food availability (summer). Hitherto it was unknown if growing king penguin chicks, in contrast to fasting adults, employed heterothermy as an extra energy-sparing mechanism when facing food shortage and harsh weather in their natural environment. Here to investigate the occurrence and determinants of heterothermy, we recorded T b of free-ranging king penguin chicks in different body sites from the deep core to the periphery ( Supplementary Fig. S1 ) over a period of up to 7 months. Variation in T b was then modelled in relation to physiological state (growth phase, nutritional condition) and several climate variables potentially influencing heat balance (air temperature, wind speed, solar radiation, rainfall). We found marked T b declines associated with physiological state, cold meals and adverse weather, a finding unexpected for large birds. Heterothermy can provide an important mechanism for king penguins to conserve energy during a long period of growth in a harsh climate and being confronted with intermittent long-term fasts. Occurrence of heterothermy T b declined gradually from the deep core near the heart ( T thorax ) towards upper abdomen ( T liver ), lower abdomen ( T lowabdo ) and the body shell ( T subcut ). 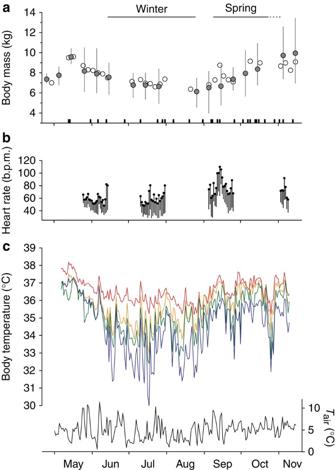Figure 1: Seasonal physiology dynamics in king penguin chicks. In panel (a) filled circles and error bars refer to 10-day body mass means and range, respectively, of ten chicks. Open circles depict individual mass for one representative chick (L7) for which feeding days are indicated by black marks at bottom of panela(feeding recordings started with first marker mid May). In panel (b) daily mean and minimum heart rate (in beats per minute) are presented for chick L7. In panel (c), daily means ofTthorax(red),Tliver(orange),Tlowabdo(green) andTsubcut(blue) are presented for the same chick (L7). Daily mean air temperature is plotted at bottom of panelc(right axis). Growth phases 'winter' and 'spring' as distinguished in the analyticalTbmodels are indicated in top of panela. The gradient between T thorax and T subcut was 1.6 °C on average during normothermia, but it can be as large as 15.7 °C (measured over 1 h; Table 1 ). Hourly T b ranged from 19 to 41 °C over all measured body sites and was most variable in the lower abdomen. Large T b declines occurred in all measured body sites including the thorax, where individual 24-h mean temperature fell as low as 33.3 °C, that is, 4.5 °C lower than normothermic T b ( Table 1 ). Prolonged T b reductions were evident throughout the winter fast, commencing when body stores were still large ( Fig. 1 ). Table 1 ∣ Body site-specific T b (°C) variation in king penguin chicks. Full size table Figure 1: Seasonal physiology dynamics in king penguin chicks. In panel ( a ) filled circles and error bars refer to 10-day body mass means and range, respectively, of ten chicks. Open circles depict individual mass for one representative chick (L7) for which feeding days are indicated by black marks at bottom of panel a (feeding recordings started with first marker mid May). In panel ( b ) daily mean and minimum heart rate (in beats per minute) are presented for chick L7. In panel ( c ), daily means of T thorax (red), T liver (orange), T lowabdo (green) and T subcut (blue) are presented for the same chick (L7). Daily mean air temperature is plotted at bottom of panel c (right axis). Growth phases 'winter' and 'spring' as distinguished in the analytical T b models are indicated in top of panel a . Full size image Heterothermy also occurred during the intensive refeeding period in spring, albeit for shorter durations ( Figs 1 and 2 ). In numerous cases, intake of cold meals regurgitated by feeding parents was associated with a profound temperature drop in stomach ( T stom ), by as much as 20 °C, and in other body sites ( Fig. 2 , event §; Supplementary Fig. S2 ). Chicks can receive more than 3 kg of food in one feeding session [9] ; therefore, heating cold food to T b may take several hours. Furthermore, heavy rainfall leading to wet down and, presumably, loss of thermal insulation could be associated with these heterothermic events ( Fig. 2 , events † and ‡). Coincidence of strong rainfall and feeding events amplified T b declines ( Fig. 2 , event ‡). 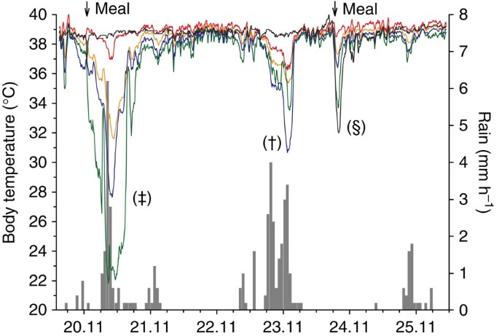Figure 2: Heterothermy induced by adverse weather and feeding in a king penguin chick. Body temperature fluctuations as measured asTthorax(red),Tliver(orange),Tlowabdo(green),Tsubcut(blue) andTstom(black) are shown for one chick (M8) during 20–25 November. Also shown are hourly rainfall (bars, right axis) and feeding events (arrows at top). Note the internal cold load in the stomach, when the chick was fed a cool meal (§) in contrast to external cooling from intensive and prolonged rainfall († and ‡). For instance, during an intensive feeding bout within a period of prolonged rainfall, one chick showed average T stom and T lowabdo of 21.1 and 19.7 °C, respectively, over a period of 13 h. Figure 2: Heterothermy induced by adverse weather and feeding in a king penguin chick. Body temperature fluctuations as measured as T thorax (red), T liver (orange), T lowabdo (green), T subcut (blue) and T stom (black) are shown for one chick (M8) during 20–25 November. Also shown are hourly rainfall (bars, right axis) and feeding events (arrows at top). Note the internal cold load in the stomach, when the chick was fed a cool meal (§) in contrast to external cooling from intensive and prolonged rainfall († and ‡). Full size image Modelling body temperature variation Although ingestion of cold meals induced occasionally very strong temperature declines in stomach and other body sites, the general effect of feeding on T b was highly variable, presumably as consequence of meals of largely varying volume and temperature ( Supplementary Fig. S2 ). Therefore, meal days were excluded from the quantitative T b models investigating determinants of heterothermy other than food temperature. This analysis revealed effects of both growth phase (season) and nutritional condition (fasting duration) as well as their interaction. T b was regulated at considerably lower level in winter compared with spring, but showed hardly any further decline related to fasting duration. In contrast, T b in spring showed significant fasting-induced declines while maintained at higher average level ( Fig. 3a ; Supplementary Table S2 ). Effects of physiological state on T b were evident in all measured body sites, but increased in magnitude with distance from the body core, reaffirming the impression from Figure 1 . As a result, the normothermic core volume was reduced and the gradient T thorax – T subcut enlarged in winter compared with spring, while accounting for possible climate effects ( Fig. 3a ; Supplementary Table S2 ). 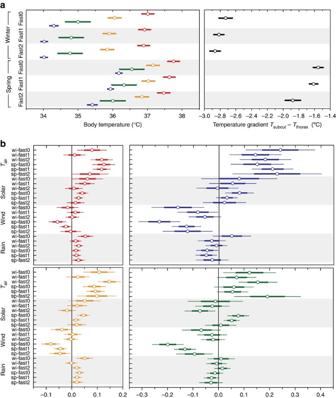Figure 3: Modelling body temperature variation in king penguin chicks. Tbestimates modelled from hourly values (n=17,279) of 10 chicks refer to means (circles), standard errors (thick bars), 95% confidence intervals (thin bars, in panelbonly) of group effects according to growth phase and nutritional condition (a) and their interactions with the climate variables ambient temperature, solar radiation, wind speed and rainfall (b); wi, 'winter'; sp, 'spring'.Tbestimates are presented for four body sites:Tthorax(red),Tliver(orange),Tlowabdo(green),Tsubcut(blue), and the gradientTsubcut−Tthorax(black, in panelaonly); for climate effects on the gradientTsubcut−TthoraxseeSupplementary Figure S3. Climate covariates were z-transformed before analyses yielding standardized slopes (b) and group mean estimates at average climate conditions (a). This allows direct comparison of effect sizes among different climate variables and amongTbfrom different body sites. Standardized slopes represent changes inTb(°C) caused by an increase of 1 standard deviation in the respective climate variable whereas other variables are held at their means. Slopes are significantly different from zero atα=0.05 (t-test), if their 95% confidence intervals do not overlap with the vertical line. Means and standard deviations of climate variables are given inSupplementary Table S1.Post-hoccomparisons of group means are listed inSupplementary Table S2. Figure 3: Modelling body temperature variation in king penguin chicks. T b estimates modelled from hourly values ( n =17,279) of 10 chicks refer to means (circles), standard errors (thick bars), 95% confidence intervals (thin bars, in panel b only) of group effects according to growth phase and nutritional condition ( a ) and their interactions with the climate variables ambient temperature, solar radiation, wind speed and rainfall ( b ); wi, 'winter'; sp, 'spring'. T b estimates are presented for four body sites: T thorax (red), T liver (orange), T lowabdo (green), T subcut (blue), and the gradient T subcut − T thorax (black, in panel a only); for climate effects on the gradient T subcut − T thorax see Supplementary Figure S3 . Climate covariates were z-transformed before analyses yielding standardized slopes ( b ) and group mean estimates at average climate conditions ( a ). This allows direct comparison of effect sizes among different climate variables and among T b from different body sites. Standardized slopes represent changes in T b (°C) caused by an increase of 1 standard deviation in the respective climate variable whereas other variables are held at their means. Slopes are significantly different from zero at α =0.05 ( t -test), if their 95% confidence intervals do not overlap with the vertical line. Means and standard deviations of climate variables are given in Supplementary Table S1 . Post-hoc comparisons of group means are listed in Supplementary Table S2 . Full size image Among climate variables, air temperature ( T air ) and wind speed had generally the strongest positive and negative influence on T b variation, respectively ( Fig. 3b ). Solar radiation and rainfall showed only relatively small average effects, when significant. Apparently, it requires extreme rainfall events to cause large T b declines extending into the body core as illustrated in Figure 2 . Climate effects on T b usually weakened from body shell to core, thereby changing the gradient T thorax – T subcut ( Fig. 3b ; Supplementary Fig. S3 ). However, T b did not always change in the same direction for all body sites. For instance, T subcut declined with increasing rainfall for certain physiological states, whereas T thorax and T liver tended to increase. Furthermore, T b responses to climate conditions varied largely depending on physiological state. For example, both T liver and T lowabdo declined significantly and, for all fasting states, with increasing wind speed in 'spring' but not in 'winter' ( Fig. 3b ). Apparently, when T b is already regulated at relatively low level as during the 'winter' stage, chicks defend this level against a further decrease, potentially caused by convective heat loss. Previous studies on the ontogeny of thermoregulation in king penguins were restricted to short-term records on restrained animals taken from the colony to the laboratory for measurement, and they concluded that T b after thermal independence (1 month from hatch) remains stable until moult [8] . In contrast, our study on unrestrained free-ranging individuals revealed pronounced T b variation both within the body and over time. This highlights the importance of studying free-living animals in their natural habitat to reveal their full behavioural and physiological repertoire [15] . The large T b gradients we observed frequently between thorax and abdomen (particularly T lowabdo ) highlight further that intraperitoneal temperatures, which are typically measured as proxies for core T b in many studies, may severely misrepresent deeper core T b ( T thorax ) in large endotherms. Many bird species respond to fasting with heterothermy [1] . Part of the T b decline during the initial stage of fasting might be attributed to reduced rates of diet-induced thermogenesis and the cessation of enzyme activity within digestive tissue. However, this effect vanishes quickly after feeding and, certainly before, end of phase I of fast [16] . Our results support previous notions that downregulation of T b can occur independently of the actual volume of body stores, and serve as an adaptive response in anticipation of energetic bottlenecks [17] . In contrast to notable metabolic changes related to fasting state in king penguins [7] , [10] , [11] , [12] , the chicks' T b showed relatively little response to nutritional condition. Seasonal effects on T b variation were much stronger. Particularly in winter, king penguin chicks defended an already low T b against further declines, despite prolonged fasting during that season. As metabolism and growth have been shown to be positively related in other avian studies [18] , metabolic constraints in growing king penguins during spring may not be compatible with regulating T b at such low levels as during the slow-down of growth in winter. On the other hand, food-restricted European shag nestlings ( Phalacrocorax aristotelis ) were able to reduce T b and metabolic rate (MR) while maintaining a high structural growth rate [19] . This suggests that heterothermy is not merely the consequence of slowed growth and reduced MR, but that T b can be regulated, to some extent, independently of these metabolic responses. Although reductions in MR may be initiated by other factors than T b declines, there is a positive feedback loop between MR and T b due to the temperature dependence of MR (Q 10 effect). Thus, as long as heat loss does not increase concomitantly, the observed reductions in normothermic core volume and downregulation of core T b in king penguin chicks indicate a reduced investment in heat production. Further energy savings can be expected from the relatively larger declines in peripheral T b that decrease heat flow between body core and shell and, if insulation of plumage is not compromised, will reduce heat loss to the environment. We argue that the combined resulting energy savings contribute markedly to the astonishing fasting capacity of king penguin chicks. A quantification of energy savings based on T b changes alone is difficult, but in the nearest species, the emperor penguin, a core temperature decrease of only 1 °C has been suggested to represent a metabolic reduction of up to 17% [20] . Supposed energy savings in king penguin chicks are further indicated by heart rate records from a concurrent study (G.E. and R.G., unpublished data) as illustrated in Figure 1 . Although calibration studies are required before we can finally quantify energy expenditure from heart rate records, our data show that heart rate largely follows T b variation. Both daily mean and daily minimum heart rate were reduced during fasting periods, and particularly in winter ( Fig. 1 ). Some of the strongest T b declines we observed were associated with the ingestion of cold meals. The reason why parents do not warm systematically the food before regurgitating it to their chick is not clear, but it is likely related to the length of the preceding foraging trip and the time delay between arrival from sea and chick-feeding. Temperature in abdomen and stomach decreases progressively with the length of a foraging trip [6] . Parents may first feed and digest for themselves but then continue to store (cold) food for the chick until the end of a foraging trip while suppressing digestion [21] . Consequently, warming of stomach content may take considerable time after arrival from sea, especially if warming occurs without digestion and only passively by the surrounding tissues, which themselves require some time for re-warming. By delivering cold meals, king penguin parents pass part of the warming cost of food on to their chick. How significant is this energetic cost for the chick? Battam and co-workers [16] quantified three major components of postprandial rise in metabolic rate (PPMR) in albatrosses after ingestion of cold meals (meal sizes were ∼ 20% of body mass): specific dynamic action (SDA), thermogenic costs of heating cold food, and thermogenic overcompensation. SDA from food at T b elevated PPMR to 4.2% of assimilated energy, whereas cold meals of 20 °C elevated PPMR to 7.7% of assimilated energy, implying certain costs of food warming and thermogenic overcompensation. Importantly, however, SDA contributed up to about 40% to the warming cost of meals (of 20 °C) from which it was generated, and this contribution will increase with higher food temperature, larger meals and longer digestion times. King penguin parents feed their chick meals that can be substantially larger than 20% of body mass, and they feed the chick slowly during sessions that may last several hours [9] . This extends the time available for SDA-generated heat to contribute to meal warming. Cost of thermogenic overcompensation may result from a marked and rapid thermoregulatory response to counter a T b decline induced by cold food [16] . However, by their heterothermic response, king penguin chicks might have largely avoided this cost. Thus, altogether, we expect food warming costs to be of little relevance to the chick's energy budget. In contrast to an active downregulation of T b as consequence of food scarcity and/or slowdown of growth, climate-induced heterothermy might be largely explained by a passive response to external factors influencing heat balance. Here the chicks can save energy by avoiding active re-warming and thermoregulation through extra heat production during episodes of adverse weather. The analysis of climate effects modelled for different physiological states indicates that the chicks allow this passive cooling only to some extent, and that they counteract heat loss to avoid a further decline in T b when already regulated at low level. Also, the finding that rainfall can induce a decline in T subcut but an increase in core T b at the same time presumably reflects some degree of active re-warming to compensate for increased heat loss due to loss of insulation when wet. To limit overall model complexity and to facilitate comparison of climate effects on T b , only their linear effects were modelled, thereby ignoring possible nonlinear responses to climate variation. For instance, it is possible that T b changes more rapidly after rainfall intensity reached a certain threshold. Also, the effects of several climate variables may not combine in a simple additive manner. For example, generally, wind can enhance heat loss but also heat gain, which will depend on T air relative to animal surface temperature. Because T air was lower than surface temperature in all measurements, our model identified the effects of convective heat loss and concomitant decrease in T b . Two of the investigated climate variables, solar radiation and T air , vary largely and periodically on a diel basis. This makes it difficult to assess their direct thermal effects on overall T b variation, because covarying T b might also be related to diel variation of other variables influencing T b (for example, activity levels) and/or have an endogenous basis. If we account for an assumed climate-independent diel T b variation in our models, the effects diminish for T air and vanish completely for solar radiation ( Supplementary Fig. S4 ). This would mean, for instance, for a given time of the day sunny or overcast weather makes no difference to T b , everything else being equal. However, it does not rule out any possible influence of solar radiation on T b differences within the 24-h period (for example, day–night differences), be it direct thermal effects or indirect effects by triggering endogenous T b rhythms. Furthermore, it is also possible that solar conditions do affect heat balance, but that compensatory thermogenesis leaves T b unchanged. Future controlled experiments may solve co-linearity problems and disentangle thermal and indirect effects of solar radiation and T air on T b patterns. By their large size, round shape, high thermal insulation of the down and thick subcutaneous fat layer, king penguin chicks are morphologically well adapted to harsh environmental conditions, which is evidenced by their having one of the lowest thermal conductance rates (0.93 Wm −2 °C −1 ) measured in large birds [22] . Pronounced heterothermy as shown in the present field study provides an extra mechanism to further reduce heat losses to a cold environment and better ensure that these birds conserve energy during a long period of growth under adverse weather conditions. Furthermore, because chicks are fully dependent on parental provisioning, their pattern of relaxed thermoregulation is not constrained by the need to be intermittently active to forage. Why, then, do they not display deeper T b declines or occasional bouts of torpor to achieve even higher energy savings during these protracted fasts? Reduced responsiveness to external stimuli makes a torpid animal vulnerable to predation, and king penguin chicks, which do not hide, cannot afford to be in a lethargic state because giant petrels ( Macronectes spec. ) patrol day and night preying on weak-looking and inattentive individuals [23] . Already a small drop in T b , not leading to a torpid state, can impair physiological and behavioural performance including predator avoidance. Thermosensitivity of muscular performance likely has a central role in shaping costs and benefits, and thereby the degree, of heterothermy in king penguin chicks [24] , [25] . Aggregation of chicks into crèches alleviates disturbance from predators and adult conspecifics, thereby allowing longer and deeper resting phases [26] that will facilitate a heterothermic stage [27] . Thus, rather than an ameliorated microclimate as observed in emperor penguin huddles [4] , [28] and suggested for adélie penguin ( Pygoscelis adeliae ) crèches [29] it could be the better sleep that represents the key energetic benefit of aggregations for king penguin chicks. Heterothermy as an energy-saving physiological response seems particular important for young dependent penguins, having little behavioural means of balancing their energy budgets. Adult penguins' long-term fasts ashore, however, are associated with either incubation or moult, and both tasks seem to constrain heterothermy [4] , [5] , [30] (but, see ref. 31 ). It would be interesting to test experimentally if fasting adults also become heterothermic once these constraints are removed. Study area The study was carried out in the Baie du Marin breeding colony ( ∼ 16,000 pairs) on Possession Island (46°25′S, 51°45′E), Crozet Archipelago, southern Indian Ocean. Average air temperature during the whole study period May–November 2008 was 5.0 °C, ranging from −3.9 to +16.5 °C. Annual rainfall in 2008 was 2,049 mm; September was the month that received most rainfall during the study period. See also Supplementary Table S1 for summary statistics of climate variables used to model T b variation. Experimental procedure and measurements All experiments were conducted on free-ranging chicks in their colony. For purposes of equipping/de-equipping birds with data loggers and for repeatedly taking measurements of body mass and size, birds were taken to a field laboratory at about 50 m distance. The experimental protocol was approved by the ethics committee of the French Polar Institute and by the French Ministry of the Environment. Authorization to enter the colony and to handle birds was obtained from Terres Australes et Antarctiques Françaises (permit No 2007-148). In late April–early May 2008, 10 birds (3–4 months old, weighing 7.0–8.6 kg, sex unknown) were equipped with 2 data loggers, each containing 3 temperature sensors: 1 inside the logger case plus 2 semi-rigid probes extending from the logger. The sensors were positioned in the thorax (near the heart, T thorax ), upper abdomen (at the liver, T liver ), lower abdomen ( T lowabdo ) and between subcutaneous fat and skin (mean of 3 sensors in ventrolateral region, T subcut ); for exact positions and anatomy, see Supplementary Figure S1 . Loggers were encased in epoxy resin, and then coated first with a layer of pasteurized wax and subsequently with a layer of medical-grade silicone (Med1137, Nusil Technology). Dimensions (W*H*L) of the logger placed subcutaneously were 15mm×40mm×30 mm, weighing 27 g. Dimensions of the logger in the abdominal cavity were 15mm×50mm×30 mm, weighing 33 g. The two probes extending from each of the loggers were 50–70 mm long and 1.5 mm in diameter. Time constants of coated sensors inside the logger case and of sensors in the external probes were 60 and 10 s, respectively. Temperature range, accuracy and sampling interval of all sensors were 0–50 °C, ±0.1 °C and 20 s, respectively. A memory capacity of 8 megabytes allowed recording for up to 300 days. Loggers were developed and manufactured within our institute. Surgeries were performed under isoflurane anesthesia. General aspects of the surgical procedure can be found elsewhere [32] . Details specific to our surgical procedure are given briefly here. Implantation of loggers was made through a first incision (perpendicular to the body axis) at the top of the 'brood patch' (a bare patch is already visible in chicks) followed by a second incision (perpendicular to the first one) of the abdominal wall. The abdominal logger was inserted into the abdominal cavity between sternum and liver and was sutured to the cartilaginous caudal end of the sternum, after the two extending probes were put in place. The subcutaneous logger was inserted between subcutaneous fat and skin, and sutured to the inner side of the skin (dermis); the two probes were tunnelled under the skin towards the flank and the brood patch. All loggers were removed surgically from all 10 chicks in late November to early December 2008, ∼ 7 months after implantation. Temperature sensors were calibrated (±0.1 °C) before and after the experiment. Data from sensors in thorax ( T thorax ) and upper abdomen ( T liver ) were successfully retrieved for all ten birds over the entire study period. In the lower abdomen ( T lowabdo ) data over the entire study period were obtained from all birds but from one; its sensor stopped recording by end of August, therefore excluding the spring period. One of the subcutaneous loggers failed downloading any data and from another subcutaneous logger data from all 3 sensors were obtained only until August. Occasionally, T subcut was unusually elevated for the first days up to few weeks after surgery, which we attribute to inflammatory processes at the place of incision. We discarded those data from quantitative analyses (for example, T subcut during May in Fig. 1 ). Stomach temperature was measured with 6mm×17 mm pill-shaped Thermochron i-buttons (model DS1922L, Dallas Semiconductor) force fed to the chicks. The logger was connected to a string with the other end glued to the feathers beneath the bill for later retrieval. Stomach temperature (±0.01 °C) was recorded each 2 min for a duration of 4–12 days per chick in the second half of November. Air temperature (±0.1 °C) and wind speed (±0.1 m s −1 ) were recorded in the colony by an automated weather station (Vantage Pro 2, Davis Instruments) at 1-min intervals. Hourly data on solar radiation (±1 J h −1 cm −2 ) and rainfall (±0.1 mm) were collected by the national weather station Alfred Faure operating at 0.9 km from the colony and obtained from Météo France. Body mass was measured with an electronic platform scale (model ITS 60K2 LIP, Kern & Sohn GmbH) to the nearest 1 g on 32–36 occasions per chick during March to November. Timing of feeding of study chicks was determined from direct observations of feeding parents and also from the relative changes in chicks' abdominal profile. Owing to infrequent but large meals, the chicks' abdomen appears notably bulged after feeding. Abdominal profiles were visually recorded on a seven-point scale every morning and evening, hence timing of feeding could be deduced at ±0.5 day resolution. As part of a concurrent study by G.E. and R.G., heart rate was recorded during four measurement periods spread over the T b study period ( Fig. 1b ) using a Polar RS 800 heart rate logger system (Polar Electro Oy) with a programmed sampling time of 5 s. For further details, including (external) attachment of devices, see Groscolas et al . [33] Data analysis Purpose-written software in Matlab (R2008b) was used for initial data treatment and exploration, including correction for linear drift in T b data, if this was indicated by comparison of pre- and post-experimental calibration. Data gathered during handling of birds were discarded from any analysis. T b variation was investigated in relation to three nutritional conditions (time since last meal) and two growth phases combining to six physiological states. Nutritional conditions can be associated with: not fasting ('fast0', 1 day postfeeding), phase I of fast ('fast1', 2–4 days postfeeding) and phase II of fast ('fast2', > 4 days postfeeding) in king penguin chicks [12] . Fuel metabolism changes towards increased fat mobilization and reduced protein utilization during phase I of fast, and protein utilization remains low throughout phase II of fast. Growth phases refer to the period from 15 June until 31 August ('winter') and the period from 16 September until moult onset ('spring'). Effect sizes of T air , wind speed, solar radiation and rainfall were modelled in interaction with physiological state. We defined 'normothermia' as reference T b based on the T b model estimates for non-fasting growing chicks ('spring-fast0') estimated for average climate conditions. T b variation was modelled with hourly values, hence all variables with originally higher sampling rate were averaged accordingly before analysis. However, rainfall was taken as the sum over two hours, over the given and previous one hour, with the reasoning that an important effect of rainfall was a wet downy plumage, which continued to last usually by roughly an hour beyond the end of rainfall. Missing value analysis revealed 4.5% missing values that would lead to 26% loss of cases if ignored in further analysis (using listwise deletion). More importantly, data were not missing completely at random (Little's MCAR test: χ 2 =4022, df=151, P <0.001) and preliminary analysis from T b models suggested non-random data loss. To avoid bias in parameter estimates [34] the multiple imputation procedure in SPSS was applied to produce three new data sets without missing values. T b models were run on these multiple data sets from which pooled estimates are presented. T b models were constructed as linear mixed-effect models including chick identity as random intercept and a first-order autoregressive covariance structure to account for serial dependency of repeated measurements ( n =1,344–2,256 per chick) within individuals ( N =10 chicks; n =17,279 in total). Fixed effects included the 'treatment' physiological state (6 levels) and its interaction with four climate covariates (air temperature, wind speed, solar radiation and rainfall). Fixed effect intercept and covariate main effects were removed from the model to allow extraction of treatment means and covariate slopes and their standard errors directly from the model output [35] . Climate covariates were z-transformed before analyses (centred to mean and divided by 1 standard deviation) yielding estimates of standardized slopes that can be compared in magnitude within models as well as between studies [35] . Presented model results were computed in the R statistical environment (version 2.12.0) using the lme-function and glht-function (Tukey's multiple comparison tests), but results were confirmed with SPSS 18. How to cite this article: Eichhorn, G. et al . Heterothermy in growing king penguins. Nat. Commun. 2:435 doi: 10.1038/ncomms1436 (2011).